A role for sorting nexin 27 in AMPA receptor trafficking Sorting nexin 27 (SNX27), a PDZ domain-containing endosomal protein, was recently shown to modulate glutamate receptor recycling in Down’s syndrome. However, the precise molecular role of SNX27 in GluA1 trafficking is unclear. Here we report that SNX27 is enriched in dendrites and spines, along with recycling endosomes. Significantly, the mobilization of SNX27 along with recycling endosomes into spines was observed. Mechanistically, SNX27 interacts with K-ras GTPase via the RA domain; and following chemical LTP stimuli, K-ras is recruited to SNX27-enriched endosomes through a Ca 2+ /CaM-dependent mechanism, which in turn drives the synaptic delivery of homomeric GluA1 receptors. Impairment of SNX27 prevents LTP and associated trafficking of AMPARs. These results demonstrate a role for SNX27 in neuronal plasticity, provide a molecular explanation for the K-ras signal during LTP and identify SNX27 as the PDZ-containing molecular linker that couples the plasticity stimuli to the delivery of postsynaptic cargo. Among over 50 Phox (PX)-domain-containing proteins in mammals, SNX27 is unique as it contains a Type I PDZ domain [1] , which is commonly found in scaffolding proteins of the postsynaptic density and junctional complexes. Most recently, it was reported that SNX27 interacts with ionotropic glutamate receptors through its PDZ domain and a reduction in SNX27 level led to synaptic dysfunction [2] . Significantly, a marked reduction in SNX27 levels was found in Down’s syndrome patients [2] . Interestingly, overexpression of miR-155, a chromosome 21-encoded microRNA negatively regulates C/EBPβ, a transcription factor regulating expression for SNX27 gene, thereby leading to a drop in SNX27 levels [2] . Despite this important discovery, the precise role of dendritic SNX27 in glutamate receptor trafficking is unknown. In addition to PDZ domain, SNX27 contains a ‘FERM-like’ domain, which consists of the F1, F2 and F3 subdomains; of which, the F1 domain was originally identified as a Ras-binding RA domain [3] . One non-canonical role of Ras is that of a signalling molecule in central synapses where it controls AMPAR trafficking during LTP. Importantly, Ras has been shown to mediate the NMDA receptor-dependent synaptic delivery of AMPARs during LTP, whereas rap mediates the NMDA receptor-dependent removal of synaptic AMPARs during long-term depression (LTD) [4] . More recent biochemical and molecular studies suggest that Ras could relay the plasticity signal into spines during LTP since recruitment of K-ras by Ca 2+ /Calmodulin (CaM) results in the translocation of K-ras from the cell membrane to early/recycling endosomes [5] . Moreover, the Ras/MAPK pathway has been linked to synaptic plasticity and memory [6] , [7] . In fact, a recent focus in LTP studies is to determine how the Ras signal leads to the synaptic delivery of AMPARs, as well as to determine what machinery directly relays the Ras signal to AMPA receptors. Since the PX domain (a phosphatidylinositol-3-phosphate (PI3P) binding domain) of SNX27 targets it to endosomes [8] , [9] , and recycling endosomes are the source of AMPARs during LTP [10] , we hypothesize that Ca 2+ influx during neuronal activity drives the recruitment of K-ras to SNX27, which in turn triggers the delivery of AMPARs to the postsynaptic surface. We have previously generated SNX27 knockout mice by inserting a neo-cassette into the third coding exon of SNX27 gene and demonstrated growth and developmental retardation with the loss of function of SNX27 (ref. 8 ). In this study, we investigate the pathological changes in the brain due to the disruption of the SNX27 gene, the distribution and mobilization of SNX27 in neurons and the functional significance of SNX27 in synaptic plasticity. Disruption of SNX27 led to hydrocephalus, pyramidal neuronal vacuolation and thinned dentate gyrus, suggesting a role for SNX27 in learning and memory. Interestingly, SNX27 is localized along with recycling endosomes in dendrites and spines. Using real-time live-cell imaging, we demonstrate the mobilization of SNX27 along with recycling endosomes into spines. We also show that SNX27 interacts with K-ras via the RA domain, and following chemical LTP stimuli, K-ras is recruited to SNX27-enriched endosomes through a Ca 2+ /CaM-dependent mechanism, which in turn drives the synaptic delivery of homomeric GluA1 receptors. Further, absence of SNX27 impairs LTP and associated trafficking of AMPARs. These results demonstrate a novel role for SNX27 in neuronal plasticity, provide a molecular explanation for the K-ras signal during LTP and identify SNX27 as the PDZ-containing molecular linker that couples the plasticity stimuli to the delivery of postsynaptic cargo. SNX27 disruption results in hydrocephalus All homozygous SNX27−/− mice are smaller, weaker, have dome-shaped heads of varying severity and display abnormal behaviours compared with their wild-type littermates. Grossly, the brains from SNX27-deficient mice were evidently pale and displayed accumulation of cerebrospinal fluid in the lateral ventricles, which collapsed upon cut ( Fig. 1a,b , Supplementary Fig. 1 ). Histological examination revealed variable degrees of bilateral dilatation of lateral ventricles, reduced thickness of cerebral cortex and dissociation of periventricular neuropil ( Fig. 1a,b ). The other major notable changes were seen in the hippocampus, which displayed vacuolation of the neuropil and CA1 and CA2 pyramidal neurons, ( Fig. 1c ) and thinning of dentate gyrus layer ( Fig. 1d ). Strikingly, quantification of the dentate gyrus layer showed that the thickness was reduced by ~30% compared with WT. 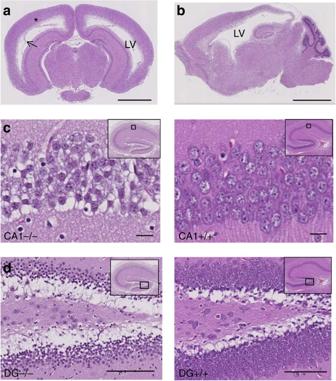Figure 1: Histopathological changes in the SNX27−/− brain. (a) Representative coronal brain section from SNX27−/− mouse stained with haematoxylin and eosin (H&E). There was dilatation of the lateral ventricle (LV), periventricular neuropil dissociation (arrow) with a rim of cortical tissue at the periphery (asterisk). Scale bar, 2 mm (b) Representative saggital sections from SNX27−/− brain stained with H&E. Scale bar, 3 mm. (c) Hippocampal CA1 region from SNX27−/− and WT mice (left and right panels, respectively). Inset shows region where the images were obtained. Scale bar, 40 μm. (d) Hippocampal dentate gyrus(DG) from SNX27−/− and WT mice (left and right panels respectively). Notable features include vacuolation of pyramidal neurons, thinning of dentate gyrus layer and cytoplasmic vacuolation. Inset shows region where the images were obtained. Scale bar, 100 μm. Figure 1: Histopathological changes in the SNX27−/− brain. ( a ) Representative coronal brain section from SNX27−/− mouse stained with haematoxylin and eosin (H&E). There was dilatation of the lateral ventricle (LV), periventricular neuropil dissociation (arrow) with a rim of cortical tissue at the periphery (asterisk). Scale bar, 2 mm ( b ) Representative saggital sections from SNX27−/− brain stained with H&E. Scale bar, 3 mm. ( c ) Hippocampal CA1 region from SNX27−/− and WT mice (left and right panels, respectively). Inset shows region where the images were obtained. Scale bar, 40 μm. ( d ) Hippocampal dentate gyrus(DG) from SNX27−/− and WT mice (left and right panels respectively). Notable features include vacuolation of pyramidal neurons, thinning of dentate gyrus layer and cytoplasmic vacuolation. Inset shows region where the images were obtained. Scale bar, 100 μm. Full size image Spine distribution of SNX27 Since histopathological data suggest that SNX27 could be important for normal hippocampal function and SNX27 contains a PDZ domain, a protein-interaction domain commonly found in scaffolding proteins of the postsynaptic density, we investigated whether SNX27 could be present in spines. To examine the distribution of SNX27 in dendrites and spines, we co-transfected cultured hippocampal neurons (17 DIV) with green fluorescent protein (GFP)-tagged SNX27 and mCherry-tagged PSD95; SNX27 was found to be enriched within or at the base of dendritic spines ( Fig. 2a ) with ~75% of spines being positive for SNX27. To verify the spine distribution of SNX27, we co-stained hippocampal neurons (15 DIV) with SNX27 and synaptophysin, a presynaptic marker. We observed the juxtaposition of SNX27 and synaptophysin ( Fig. 2b ), further confirming the postsynaptic localization of SNX27. Tagged versions of SNX27 were verified by sequencing and comparing its expression with endogenous SNX27 protein ( Supplementary Fig. 2 ). 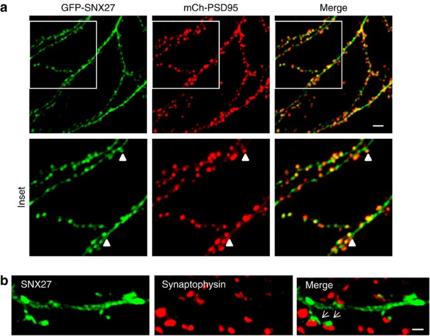Figure 2: Spine distribution of SNX27 in neurons. (a) Cultured hippocampal neurons (17 div) transfected with GFP-tagged SNX27 and mCherry-PSD95 to identify spines. SNX27 was distributed on the base of spines and within dendritic spines. Scale bar, 4 μm. (b) Cultured hippocampal neurons (17 div) transfected with GFP-tagged SNX27. Neurons were then labelled with presynaptic marker, synaptophysin. SNX27 labelling is closely opposed to that of synaptophysin (arrows). Scale bar, 1 μm. Figure 2: Spine distribution of SNX27 in neurons. ( a ) Cultured hippocampal neurons (17 div) transfected with GFP-tagged SNX27 and mCherry-PSD95 to identify spines. SNX27 was distributed on the base of spines and within dendritic spines. Scale bar, 4 μm. ( b ) Cultured hippocampal neurons (17 div) transfected with GFP-tagged SNX27. Neurons were then labelled with presynaptic marker, synaptophysin. SNX27 labelling is closely opposed to that of synaptophysin (arrows). Scale bar, 1 μm. Full size image SNX27 has three structural domains: the PDZ, PX and RA domains. To establish the role of each domain in spine distribution, we constructed three deletion mutants with each of the structural domains independently deleted: GFP-tagged SNX27ΔPDZ, SNX27ΔPX and SNX27ΔRA and verified their expression by transfecting cultured neurons (14 DIV) with the respective construct and examining their fluorescence signal ( Supplementary Fig. 3 ). For the truncated constructs, expression was limited to the cell body and proximal dendrites; little to no expression was detected in the distal dendrites and spines ( Supplementary Fig. 3 ). We further took hippocampal neurons (17 DIV), transfected them with the respective constructs and quantified the green and red fluorescence signal along the length (dashed line) of the image ( Fig. 3 ). For full-length SNX27, there is overlap of the red and green peaks indicating colocalization of the corresponding spots, whereas for the mutants, the green peaks are much lower than the red peak indicating minimal distribution in the spines. Taken together, the result demonstrates the loss of spine distribution with all three mutants and suggests the collective importance of all three structural domains for spine distribution. 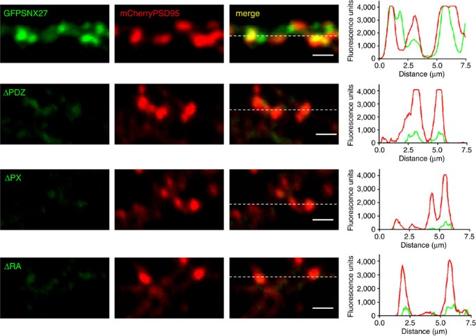Figure 3: Loss of spine distribution in the truncated mutants. Cultured hippocampal neurons (17 div) transfected with GFP-tagged full-length SNX27 or SNX27 deletion mutants. mCherry-PSD95 was also expressed to identify spines. Fluorescence signal was quantified along the length (dashed line) of the image. For full-length SNX27, there is overlap of the red and green peaks indicating colocalization of the corresponding spots, whereas for the mutants, the green peaks are much lower than the red peak indicating minimal localization in the spines. Scale bar, 2 μm. Figure 3: Loss of spine distribution in the truncated mutants. Cultured hippocampal neurons (17 div) transfected with GFP-tagged full-length SNX27 or SNX27 deletion mutants. mCherry-PSD95 was also expressed to identify spines. Fluorescence signal was quantified along the length (dashed line) of the image. For full-length SNX27, there is overlap of the red and green peaks indicating colocalization of the corresponding spots, whereas for the mutants, the green peaks are much lower than the red peak indicating minimal localization in the spines. Scale bar, 2 μm. Full size image Dynamic SNX27 clusters translocate into spines SNX27 has a PX domain crucial for interaction with phospholipid (PI3P) in endosomes, an essential source of AMPARs during LTP [10] . To examine the distribution of SNX27 in endosomes, we co-labelled hippocampal neurons (16 DIV) with early endosome marker, Rab5 and classic recycling endosome markers—transferrin receptor and Rab11—along with SNX27. We found extensive localization of SNX27 with both early and recycling endosomes ( Fig. 4a,b ). 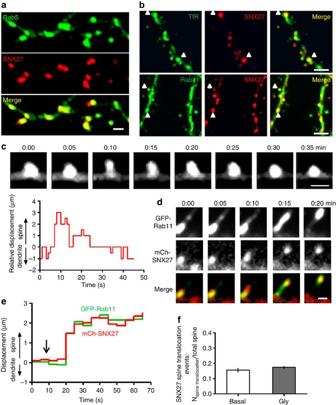Figure 4: Mobilization of SNX27 into spines along with recycling endosomes. (a) Colocalization of SNX27 with early endosomes marked by Rab5. Scale bar, 1 μm. (b) Recycling endosomes were labelled with transferrin receptor and Rab 11. Colocalization of SNX27 with recycling endosomes marked by tranferrin receptor and Rab11 as indicated with arrowheads. Scale bar, 2 μm. (c) Rapid time-lapse images of SNX27 revealing its mobilization in and out of spine (upper). Time is indicated in minutes and seconds. Step-wise displacement analysis of GFP-SNX27 puncta with base of spine defined as zero (lower). Scale bar, 1 μm. (d) Time-lapse imaging showing the mobilization of SNX27 along with recycling endosomes into spine. Time is indicated in minutes and seconds. Scale bar, 1 μm. (e) Step-wise displacement analysis showing the correlated movement of the GFP and mCherry signal ind. (f) SNX27 spine translocation events (events per min/total spine) were measured with or without glycine treatment. The graph represents the means of 15 independent experiments.n=15,P=0.2663, unpairedt-test, error bars=s.e.m. Figure 4: Mobilization of SNX27 into spines along with recycling endosomes. ( a ) Colocalization of SNX27 with early endosomes marked by Rab5. Scale bar, 1 μm. ( b ) Recycling endosomes were labelled with transferrin receptor and Rab 11. Colocalization of SNX27 with recycling endosomes marked by tranferrin receptor and Rab11 as indicated with arrowheads. Scale bar, 2 μm. ( c ) Rapid time-lapse images of SNX27 revealing its mobilization in and out of spine (upper). Time is indicated in minutes and seconds. Step-wise displacement analysis of GFP-SNX27 puncta with base of spine defined as zero (lower). Scale bar, 1 μm. ( d ) Time-lapse imaging showing the mobilization of SNX27 along with recycling endosomes into spine. Time is indicated in minutes and seconds. Scale bar, 1 μm. ( e ) Step-wise displacement analysis showing the correlated movement of the GFP and mCherry signal in d . ( f ) SNX27 spine translocation events (events per min/total spine) were measured with or without glycine treatment. The graph represents the means of 15 independent experiments. n =15, P =0.2663, unpaired t -test, error bars=s.e.m. Full size image To gain insights into the dynamics of SNX27-marked clusters, we performed rapid time-lapse imaging of GFP-SNX27-transfected hippocampal neurons. Interestingly, while in younger neurons (12 DIV), we observe the shuttling of SNX27 up and down the filipodia ( Supplementary Fig. 4a ), in older neurons (18 DIV), we observed the dynamic movements of SNX27 in and out of spines ( Fig. 4c ). In the latter, the result was quantified by charting the displacement of the fluorescent maxima with time ( Fig. 4c ). Detailed analysis showed that the vesicle travelled from the base of the spine to the spine head at a speed of up to ~0.7 μm s −1 . In fact, since recycling endosomes are dynamic cellular compartments that are mobilized into spines during LTP, we studied the correlated movement of SNX27 and recycling endosomes into spines using rapid time-lapse imaging. Interestingly, we observed the spatio-temporally correlated movement of Rab11 and SNX27 into spines following chemical LTP stimuli (glycine 200 μM; Fig. 4d,e ). Additional time-lapse images of the coordinated movement of Rab11 and SNX27 into spines are shown in Supplementary Fig. 4b . Importantly, there was no statistically significant difference in the number of SNX27 spine translocation events per min under basal condition or following glycine stimulation ( Fig. 4f ); indicating that SNX27 spine translocation events do not require chemical LTP stimulation. Loss of SNX27 from spines following chemical LTP stimulation To define the role of SNX27 for the delivery of postsynaptic cargo during synaptic plasticity, we transfected cultured neurons (18 DIV) with GFP-SNX27 and mCherry-PSD95 and followed the GFP signal before and after LTP-inducing stimuli (glycine 200 μM, 5 min). We observed the selective loss of GFP signal (~33%) from the spines with glycine stimulation, but not in the presence of APV ( Fig. 5a,b ), while the mCherry signal from PSD95 remained unchanged ( n =87 and 90 spines from five neurons for Gly and Gly/APV treatment, respectively). This result suggests that chemical LTP stimulus induces the fusion of SNX27-positive recycling endosomes with the plasma membrane and the consequent diffusion of GFP signal. Importantly, the GFP signal recovered following the washout of glycine, suggesting the reformation of SNX27-containing endosomes in the spines upon removal of the LTP stimulus ( Fig. 5a,b ). 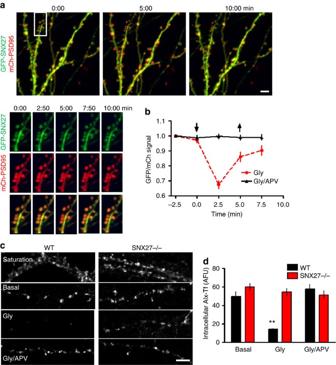Figure 5: SNX27 mediates recycling endosome transport. (a) Loss of SNX27 from spines following glycine treatment. Time-lapse imaging following the loss and subsequent recovery of SNX27 signal (green) with time following glycine treatment, but not in the presence of NMDA receptor antagonist APV. Glycine stimulation was applied from 0–5 min. Time is indicated in minutes and seconds. Scale bar, 4 μm. (b) Quatitative analysis of loss of SNX27 GFP signal normalized against the spine mcherry signal (n=87 and 90 spines from 5 neurons for Gly and Gly/APV treatment respectively, error bars=s.e.m.). (c) Absence of SNX27 interferes with recycling endosome transport. Wild type and SNX27-depleted neurons were saturated with Alx-Tf for 30 min, washed and further incubated in neurobasal media, glycine or glycine/APV for 25 min. Representative images showing the loss of Alx-Tf from wild type and SNX27-deficient neurons following 25 min treatment with neurobasal media, glycine or glycine/APV. Scale bar, 5 μm. (d) Quantitative analysis of intracellular fluorescence remaining following 25 min treatment with neurobasal media, glycine or glycine/APV;n=10 neurons respectively, error bars=s.e.m. ** indicatesP<0.05 for WT vs SNX27-/-(glycine treated), unpairedt-test. Figure 5: SNX27 mediates recycling endosome transport. ( a ) Loss of SNX27 from spines following glycine treatment. Time-lapse imaging following the loss and subsequent recovery of SNX27 signal (green) with time following glycine treatment, but not in the presence of NMDA receptor antagonist APV. Glycine stimulation was applied from 0–5 min. Time is indicated in minutes and seconds. Scale bar, 4 μm. ( b ) Quatitative analysis of loss of SNX27 GFP signal normalized against the spine mcherry signal ( n =87 and 90 spines from 5 neurons for Gly and Gly/APV treatment respectively, error bars=s.e.m.). ( c ) Absence of SNX27 interferes with recycling endosome transport. Wild type and SNX27-depleted neurons were saturated with Alx-Tf for 30 min, washed and further incubated in neurobasal media, glycine or glycine/APV for 25 min. Representative images showing the loss of Alx-Tf from wild type and SNX27-deficient neurons following 25 min treatment with neurobasal media, glycine or glycine/APV. Scale bar, 5 μm. ( d ) Quantitative analysis of intracellular fluorescence remaining following 25 min treatment with neurobasal media, glycine or glycine/APV; n =10 neurons respectively, error bars=s.e.m. ** indicates P <0.05 for WT vs SNX27-/-(glycine treated), unpaired t -test. Full size image Impaired recycling in the absence of SNX27 Cultured hippocampal neurons from SNX27 knockout mice would provide a powerful tool for testing the physiological importance of SNX27 in endosome recycling. The effect of LTP-inducing stimuli on overall endocytic recycling in SNX27-deficient neurons was measured by using fluorescently labelled transferrin, cargo of constitutive recycling. WT and knockout neurons (17 DIV) exhibited robust uptake of Alx-Tf at steady state (30 min saturation). Subsequent 25-min incubation in extracellular solution without labelled transferrin revealed some loss of intracellular Alx-Tf, reflecting ongoing basal recycling ( Fig. 5c,d ). Remarkably, brief application of LTP stimulus (glycine 200 μM) accelerated the recycling of intracellular Alx-Tf in normal neurons but not the knockouts ( Fig. 5c,d ; WT: 14.5±1.6; SNX27−/−: 52.5±10.2, mean±s.e.m., P <0.01 Student’s t -test, n =10 neurons, respectively). Furthermore, the Gly-induced increase in transferrin recycling in normal neurons was prevented by co-application of APV (100 μM), indicating a requirement for NMDA receptor activation. Since NMDA receptor activation is required in Gly-induced recycling, we need to be convinced that impaired recycling observed in the knockouts is due to the absence of SNX27 and not the result of drastic alteration in endogenous GluN1 expression in the SNX27−/− neurons. We analysed GluN1 expression levels in the hippocampus of wild type and SNX27−/− mice. Our blotting results show similar expression of GluN1 in the synaptosome and Triton-insoluble (PSD) fraction ( Fig. 6 ). Quantitative analysis showed that there was a slight decline in GluN1 expression in the synaptosome and PSD fraction of the SNX27 −/− hippocampus compared with wild type (82% and 85% respectively; n =3; P <0.05, Student’s t -test). However, it is unlikely that this small difference in GluN1 levels could account for the large impairment in transferrin recycling observed here. Therefore, we conclude that overall transferrin transport from recycling endosomes to plasma membrane is significantly compromised in SNX27-deficient neurons. 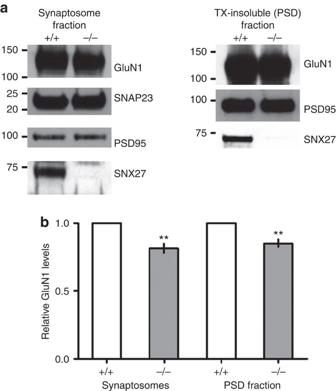Figure 6: GluN1 expression in wild type and SNX27−/− mice. (a) GluN1 amounts in synaptosomes and PSD fractions derived from wild type and SNX27−/− hippocampus. (b) Graph shows the GluN1 levels in synaptosomes and PSD fractions of SNX27−/− hippocampus relative to wild-type hippocampus.n=3; **indicatesP<0.05, unpairedt-test; error bars=s.e.m. Figure 6: GluN1 expression in wild type and SNX27−/− mice. ( a ) GluN1 amounts in synaptosomes and PSD fractions derived from wild type and SNX27−/− hippocampus. ( b ) Graph shows the GluN1 levels in synaptosomes and PSD fractions of SNX27−/− hippocampus relative to wild-type hippocampus. n =3; **indicates P <0.05, unpaired t -test; error bars=s.e.m. Full size image K-ras selectively interacts with SNX27 Since activity causes redistribution of K-ras from the plasma membrane to endosomes [7] ( Supplementary Fig. 5a ), we hypothesized that SNX27 is likely the endosome-docking molecule that decodes the plasticity signal from K-ras and drives GluA1 receptors into spines. To determine the K-ras-binding properties of SNX27, coimmunoprecipitation with anti-SNX27 was performed. K-ras (but not H-ras or N-ras) selectively interacts with SNX27 on endogenous hippocampal lysate ( Fig. 7a ). To validate this interaction, we expressed HA-K-ras and either myc-SNX27 or myc-SNX27-lacking K-ras-binding (RA) domain in HEK cells and immunoprecipitated with myc-antibody. As expected, full-length SNX27 ( Fig. 7a , lower panel; lane 3) but not the truncated SNX27 (lane 4) interacted with K-ras, indicating that the SNX27 RA domain is required for the interaction with K-ras. 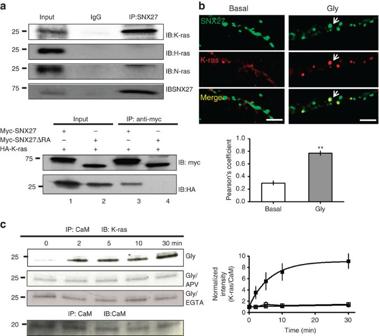Figure 7: Ras-binding properties of SNX27. (a) Upper panel: selective interaction of endogenous K-ras with SNX27 in hippocampal lysate. Lower panel: immunoprecipitation of HEK293 cells expressing HA-K-ras and Myc-SNX27 full-length or SNX27 lacking RA domain (Myc-SNX27ΔRA). (b) Localization of SNX27 and K-ras with and without glycine treatment (200 μm, 5 min). The graph represents the mean of five independent experiments with 10 images each. (n=5, ** indicatesP<0.05, unpairedt-test, error bars=s.e.m.). Scale bar, 2 μm. (c) Time dependence of K-ras binding to calmodulin following Gly, Gly/APV and Gly/EGTA stimulation (upper). Quantitative analysis of time course of K-ras binding to CaM following Gly (▪), Gly/APV (□) and Gly/EGTA (Δ) stimulation (lower).n=3. All error bars represent s.e.m. Figure 7: Ras-binding properties of SNX27. ( a ) Upper panel: selective interaction of endogenous K-ras with SNX27 in hippocampal lysate. Lower panel: immunoprecipitation of HEK293 cells expressing HA-K-ras and Myc-SNX27 full-length or SNX27 lacking RA domain (Myc-SNX27ΔRA). ( b ) Localization of SNX27 and K-ras with and without glycine treatment (200 μm, 5 min). The graph represents the mean of five independent experiments with 10 images each. ( n =5, ** indicates P <0.05, unpaired t -test, error bars=s.e.m.). Scale bar, 2 μm. ( c ) Time dependence of K-ras binding to calmodulin following Gly, Gly/APV and Gly/EGTA stimulation (upper). Quantitative analysis of time course of K-ras binding to CaM following Gly (▪), Gly/APV (□) and Gly/EGTA (Δ) stimulation (lower). n =3. All error bars represent s.e.m. Full size image Under resting conditions, the majority of K-ras is localized to the plasma membrane. To visualize the physical interaction of SNX27 with K-ras, we stimulated hippocampal neurons (15 DIV) with glycine (200 μM, 5 min), fixed and stained them with SNX27 and K-ras antibodies. Before glycine treatment, there was minimal colocalization of SNX27 and K-ras (Pearson’s coefficient=0.30±0.03, mean±s.e.m., n =5). After glycine stimulation, significant colocalization of SNX27 and K-ras (Pearson’s coefficient=0.77±0.04, mean±s.e.m., n =5) was observed (arrows, Fig. 7b ), indicating that activity causes the redistribution of K-ras from the plasma membrane to SNX27-containing endosomes. During synaptic potentiation, CaM is the predominant Ca 2+ sensor. Several studies have examined the selective interaction between K-ras and Ca 2+ /CaM [11] , [12] and examined the K-ras-binding state(GTP versus GDP), which we have verified and confirmed ( Supplementary Fig. 5b,c ). To establish whether Ca 2+ influx during synaptic potentiation drives the binding of CaM to K-ras, we examined the time dependence of K-ras CaM binding following chemical LTP stimulus (glycine, 200 μM) by coimmunoprecipitation. Importantly, we observed a time-dependent increase in K-ras-binding to CaM following glycine stimulus ( τ =5.9 min), which requires NMDA receptor activation and Ca 2+ , as no increase was detected with the co-application of APV (100 μM) or EGTA (3 mM) ( Fig. 7c , n =3). SNX27 interacts with GluA1 receptors via PDZ domain Synaptic accumulation of AMPARs during LTP requires interaction between GluA1 and a yet to be defined Type I PDZ domain-containing protein [13] , [14] . Therefore, we hypothesized that SNX27 interacts with GluA1 via its PDZ domain and drives AMPARs to dendritic spines following LTP. Consistent with our hypothesis, endogenous coimmunoprecipitation of endogenous proteins showed that SNX27 forms a complex with GluA1, but not GluA2 (a Type II PDZ domain interacting protein), in native hippocampal lysate ( Fig. 8a ). This interaction is independent of scaffolding proteins of the postsynaptic density (SAP97 and PSD95) ( Fig. 8a ). Since previously it was reported that SNX27 interacts with GluA2 via in vitro recombinant pull-down and coimmunoprecipitation from HEK cells [2] , we verified our endogenous immunoprecipitation results by performing a reverse endogenous coimmunoprecipitation, a highly stringent and less promiscuous method for detecting real (and most likely direct) protein interaction in vivo . Reverse co-immunoprecipitation with GluA2 antibody revealed that GluA2 interacts with GluA1, but not SNX27 ( Fig. 8b ), thus further verifying that GluA2 does not interact with SNX27. 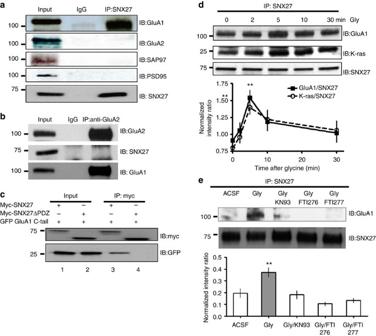Figure 8: AMPAR binding properties of SNX27. (a) Endogenous coimmunoprecipitation with SNX27 antibody. SNX27 interacts with GluA1 receptor, but not GluA2 receptor. (b) Reverse coimmunoprecipitation with GluA2 antibody to verify interaction of GluA2 with GluA1. GluA2 interacts with GluA1, but not SNX27. (c) Immunoprecipitation of HEK293 cells expressing GFP-GluA1 c-terminal tail and Myc-SNX27 or Myc-SNX27 without the PDZ domain (Myc-SNX27ΔPDZ). (d) Time dependence of enhanced K-ras and GluA1 binding to SNX27 following Gly stimulation (upper). Quantitative analysis of time course of K-ras and GluA1 binding to SNX27 following Gly stimulation (lower). The density bands at each time point for GluA1 and K-ras were normalized against the respective SNX27 density band at the same time point. This result would give the normalized intensity ratio on theyaxis and these were plotted against time on thexaxis.n=3, ** indicatesP⩽0.01, unpairedt-test; error bars=s.e.m. (e) Recruitment of GluA1 by SNX27 is inhibited by CaM kinase inhibitor (KN93) and farnesyltransferase inhibitors (FTI-276 and FTI-277). The GluA1 density bands were normalized against the respective SNX27 density band. This result would give the normalized intensity ratio on theyaxis.n=3, ** indicatesP⩽0.05, unpairedt-test; error bars=s.e.m. Figure 8: AMPAR binding properties of SNX27. ( a ) Endogenous coimmunoprecipitation with SNX27 antibody. SNX27 interacts with GluA1 receptor, but not GluA2 receptor. ( b ) Reverse coimmunoprecipitation with GluA2 antibody to verify interaction of GluA2 with GluA1. GluA2 interacts with GluA1, but not SNX27. ( c ) Immunoprecipitation of HEK293 cells expressing GFP-GluA1 c-terminal tail and Myc-SNX27 or Myc-SNX27 without the PDZ domain (Myc-SNX27ΔPDZ). ( d ) Time dependence of enhanced K-ras and GluA1 binding to SNX27 following Gly stimulation (upper). Quantitative analysis of time course of K-ras and GluA1 binding to SNX27 following Gly stimulation (lower). The density bands at each time point for GluA1 and K-ras were normalized against the respective SNX27 density band at the same time point. This result would give the normalized intensity ratio on the y axis and these were plotted against time on the x axis. n =3, ** indicates P ⩽ 0.01, unpaired t -test; error bars=s.e.m. ( e ) Recruitment of GluA1 by SNX27 is inhibited by CaM kinase inhibitor (KN93) and farnesyltransferase inhibitors (FTI-276 and FTI-277). The GluA1 density bands were normalized against the respective SNX27 density band. This result would give the normalized intensity ratio on the y axis. n =3, ** indicates P ⩽ 0.05, unpaired t -test; error bars=s.e.m. Full size image To validate the interaction between SNX27 and GluA1, we expressed GFP-GluA1 C-terminal tail with either full-length myc-SNX27 or myc-SNX27 lacking PDZ domain in HEK cells and co-immunoprecipitated with myc-antibody. As expected, GFP-GluA1 C-terminal tail was able to pull-down full-length SNX27 ( Fig. 8c , lower panel; lane 3), but not myc-SNX27ΔPDZ (lane 4), establishing that GluA1 C-terminal PDZ-binding motif is important for the interaction with SNX27 PDZ domain. Next, we examined the time dependence of SNX27/GluA1 interaction following Gly stimulation (200 μM). There was a statistically significant increase in SNX27/GluA1 binding that peaks at ~5 min ( Fig. 8d , n =3). Importantly, a corresponding increase in the levels of K-ras was detected in the pull-down with SNX27 ( Fig. 8d ), suggesting that SNX27 is likely a molecular linker that captures the plasticity signal from K-ras and links the plasticity signal to the recruitment of GluA1 AMPARs. The recruitment of GluA1 to SNX27 following glycine requires Ca/CaM as it was inhibited by KN93, a Ca/CaM-dependent protein kinase inhibitor ( Fig. 8e ). To test the role of K-ras in the recruitment of GluA1 to SNX27, we incubated cultured neurons with farnesyltransferase inhibitor FTI - 276 or FTI-277. Farnesylation attaches K-ras to the cell membrane, a step essential for the transfer of signals from membrane receptors. Overnight incubation with either FTI-276 (5 μM) or FTI-277 (5 μM) abolishes the interaction between GluA1 and SNX27, indicating that K-ras is necessary for the recruitment of GluA1 by SNX27. Although inhibitor experiments cannot exclude the involvement of other prenylated proteins, the coimmunoprecipitation experiments shown above strongly indicate that K-ras is the protein linking the plasticity signal to the recruitment of GluA1 AMPARs via Ca/CaM-dependent process. Since it was reported that SNX27 stabilizes retromer cargo proteins and SNX27 depletion led to reduced expression of retromer cargoes owing to enhanced lysosomal degradation of these proteins [15] , we determined whether SNX27 might similarly affect GluA1 levels in the knockout neurons. We found that GluA1 expression was reduced in SNX27−/− neurons ( Supplementary Fig. 6a ). Blocking lysosomal proteases with leupeptin significantly enhanced GluA1 levels in SNX27-depleted cells ( Supplementary Fig. 6b ); indicating that enhanced lysosomal degradation of GluA1, in the absence of SNX27, led to a decrease in GluA1 levels. SNX27 important for AMPA receptor delivery and LTP To determine the efficiency of GluA1 surface insertion in the absence of SNX27, time-lapse live cell imaging was performed on cultured hippocampal neurons (17 DIV) ectopically expressing superecliptic phluorin-GluA1 (SEP-GluA1). In these experiments, mCherry-PSD95 was also expressed to identify spines. For WT neurons, LTP stimulation (glycine 200 μM, 5 min) triggered a clear elevation (nearly twofold increase) in SEP-GluA1 signal in spines ( n =10 neurons, Fig. 9a,b ; Supplementary Movie 1 ). In contrast, the SEP-GluA1 signal barely increased in the absence of SNX27 ( n =10 neurons, Fig. 9a,b and Supplementary Movie 2 ). To address the possible role of GluA2 in this model of cellular plasticity, we examined the role of GluA2 in glycine-induced LTP. We expressed SEP-GluA2 in wild-type cultured hippocampal neurons (17 DIV) and assessed GluA2 surface insertion by live-cell time-lapse imaging. Our results show that there was no increase in SEP-GluA2 signal in spines following glycine application ( Supplementary Fig. 7 ), suggesting that surface insertion of GluA2 is absent in the early phase of this cellular model of LTP. We then continued to perform the same experiment on SNX27 knockout neurons and similarly, there was no increase in SEP-GluA2 signal ( Supplementary Fig. 7 ). Taken together, our results indicate that insertion of GluA1, but not GluA2, is important for synaptic plasticity following glycine-induced LTP, and SNX27 is important for the surface insertion of GluA1 receptors in cultured hippocampal neurons during chemical-induced LTP. 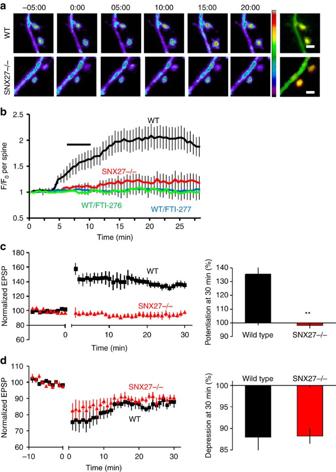Figure 9: Disrupting SNX27 interferes with AMPA receptor surface delivery and LTP. (a) Time-lapse SEP-GluA1 fluorescence images from wild type and SNX27-deficient neurons with 5 min glycine treatment. mCherry-PSD95 was used to identify spines (right-most image). Scale bar, 1 μm. (b) The normalized increase in SEP-GluA1 fluorescence (Ft/F0) in spines was monitored in wild type, wild type treated with FTI-276 and FTI-277 and SNX27-deficient neurons;n=10 neurons respectively. Bar indicates presence of glycine stimulus. (c) Hippocampal slices were freshly prepared from wild type and SNX27 knockout mice and LTP was induced using high‐frequency stimulation in normal (squares) and SNX27-deficient slices (triangles);n=8 slices respectively. Bar graph summarizing the effect of SNX27 deletion on the magnitude of LTP at 30 min (** indicatesP<0.001,t-test, error bars=s.e.m.). (d) LTD in wild type versus knockout slices with 1 Hz stimulation for 15 min;n=7 slices respectively. Bar graph summarizing the effect of SNX27 deletion on the magnitude of LTD at 30 min (P>0.9,t-test, error bars=s.e.m.). Figure 9: Disrupting SNX27 interferes with AMPA receptor surface delivery and LTP. ( a ) Time-lapse SEP-GluA1 fluorescence images from wild type and SNX27-deficient neurons with 5 min glycine treatment. mCherry-PSD95 was used to identify spines (right-most image). Scale bar, 1 μm. ( b ) The normalized increase in SEP-GluA1 fluorescence ( F t / F 0 ) in spines was monitored in wild type, wild type treated with FTI-276 and FTI-277 and SNX27-deficient neurons; n =10 neurons respectively. Bar indicates presence of glycine stimulus. ( c ) Hippocampal slices were freshly prepared from wild type and SNX27 knockout mice and LTP was induced using high‐frequency stimulation in normal (squares) and SNX27-deficient slices (triangles); n =8 slices respectively. Bar graph summarizing the effect of SNX27 deletion on the magnitude of LTP at 30 min (** indicates P <0.001, t -test, error bars=s.e.m.). ( d ) LTD in wild type versus knockout slices with 1 Hz stimulation for 15 min; n =7 slices respectively. Bar graph summarizing the effect of SNX27 deletion on the magnitude of LTD at 30 min ( P >0.9, t -test, error bars=s.e.m.). Full size image To more directly evaluate the role of SNX27 in synaptic plasticity, we induced LTP and measured field excitatory postsynaptic potentials (fEPSPs) in the Schaffer collateral pathway of acute hippocampal slices from WT and SNX27 knockout mice (4-week-old). In control slices, brief high-frequency afferent stimulation (100 Hz, 1 s) of the Schaffer collateral inputs elicited robust LTP ( Fig. 9c , n =8 slices) and the absence of SNX27 resulted in the complete loss of the LTP response ( Fig. 9c ). Analysis of degree of potentiation at 30 min ( Fig. 9c , right) confirmed the loss of LTP response in the knockout slices, thereby providing direct evidence for the role of SNX27 in synaptic potentiation. We therefore conclude that SNX27 is important for the synaptic delivery of AMPARs associated with LTP. We also investigated the possible role of SNX27 in AMPAR retrieval by examining LTD in the same Schaffer collateral pathway. In control slices, prolonged low-frequency afferent stimulation (1 Hz, 15 min) caused LTD ( Fig. 9d , n =7 slices), while disruption of SNX27 had no effect on the LTD response from the same recording site ( Fig. 6d ). Analysis of degree of synaptic depression at 30 min ( Fig. 9d , right) showed no significant difference in response between the WT and the knockout slices; this indicates that synaptic retrieval of AMPARs is unaffected by the absence of SNX27. Together, these experiments reveal that SNX27 is selectively required for AMPAR insertion associated with synaptic potentiation in living slices. Down’s syndrome, or triosmy 21, is a congenital disorder characterized by developmental delays, learning abnormalities and multiple organ defects [16] . It was recently reported that loss of SNX27 mediates excitatory synaptic dysfunction and modulates glutamate receptor recycling in Down’s syndrome [2] . However, the exact molecular mechanism by which SNX27 affects glutamate receptor recycling is unknown. This study demonstrates that during synaptic activity, SNX27 captures the calcium-triggered plasticity signal from K-ras; this initial step promotes the recruitment of GluA1 receptors to SNX27 and subsequently drives the synaptic delivery of GluA1 AMPARs ( Fig. 10 ). 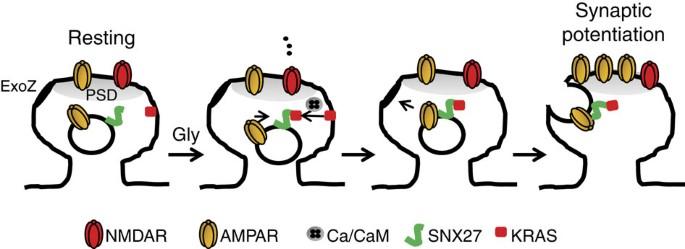Figure 10: Schematic model for LTP induction. PSD, postsynaptic density; ExoZ, exocytic zone. During synaptic activity, binding of Ca to CaM triggers the translocation of K-ras from the plasma membrane to SNX27 on recycling endosomes. This initial binding step promotes the recruitment of GluA1 receptors to SNX27 on recycling endosomes and subsequently drives the synaptic delivery of GluA1 AMPARs. Figure 10: Schematic model for LTP induction. PSD, postsynaptic density; ExoZ, exocytic zone. During synaptic activity, binding of Ca to CaM triggers the translocation of K-ras from the plasma membrane to SNX27 on recycling endosomes. This initial binding step promotes the recruitment of GluA1 receptors to SNX27 on recycling endosomes and subsequently drives the synaptic delivery of GluA1 AMPARs. Full size image Hydrocephalus is a condition characterized by excess accumulation of cerebrospinal fluid and enlargement of ventricles in the brain. Histological examination of the knockout mice revealed that mice lacking SNX27 develop congenital hydrocephalus characterized by enlarged ventricles, thinned cortex and atrophy of the periventricular white matter. A few cases of Down’s syndrome have been associated with hydrocephalus; some do not make it to term while others that survive are treated for hydrocephalus—mainly by shunting the excessive fluid [17] , [18] , [19] , [20] . It is unclear how the condition of an additional copy of chromosome 21 leads to hydrocephalus. Further investigation of the role of SNX27 in the pathogenesis of hydrocephalus in these mice may help to define the role of the extra chromosome in hydrocephalus. SNX27 contains a PX domain that selectively binds to membrane phospholipid phosphatidylinositol-3-phosphate (PI3P) on endosomes. In recent years, a number of studies have demonstrated the importance of SNX27 for endosome-to-plasma membrane trafficking; in particular, SNX27 regulates the trafficking of 5-HT4a receptor [21] , β 2 -adrenoreceptor [9] , [22] and potassium channels [23] via its PDZ domain interaction. A recent proteomics analysis further established that SNX27 is likely a general endosomal sorting protein regulating recycling of hundreds of surface proteins, many of which have C-terminal PDZ-binding motif [15] . In the present study, we showed that SNX27 is dynamically distributed on recycling endosomes in dendrites and within dendritic spines. Ablation of SNX27 in neurons strongly interfered with the endosome-to-plasma membrane trafficking of the constitutive recycling endosome cargo, transferrin, and resulted in greater retention of transferrin within the cell. This result provides clear evidence that overall transport from recycling endosomes to the plasma membrane is compromised in SNX27-deficient neurons. Since LTP is the dominant cellular model of learning and memory and recycling endosomes are an essential source of AMPARs during LTP, we examined the interaction between SNX27 and AMPA receptors. AMPA receptors are viewed as heterotetramers, contributed by the AMPAR subunits: GluA1, GluA2, GluA3 and GluA4 (ref. 24 ). However, the precise subunit composition of the AMPAR involved in LTP has been somewhat controversial [25] , [26] , [27] , [28] , [29] , [30] , [31] . While one line of evidence suggests that early LTP is mediated by the selective recruitment of homomeric GluA1 AMPARs to synapses, which are then gradually replaced by GluA2-containing AMPARs during the maintenance phase of LTP [25] , [26] , [27] , another line of evidence suggests that hippocampal LTP can take place independent of GluA1 receptors [28] , [29] and a variety of other glutamate receptor subtypes (that is, GluA2, GluK1) have the ability to potentiate synapses [30] . Brief glycine application is known to simulate the early phase of LTP. Our results showed that there was surface insertion of GluA1, but not GluA2 receptors, following brief glycine stimulation ( Fig. 9 and Supplementary Fig. 7 ). Furthermore, SNX27 specifically interacts with GluA1, but not GluA2 ( Fig. 8 ). Contrary to this result, an earlier paper demonstrated using recombinant GST-fused SNX27 and overexpression in HEK cells that SNX27 pulled down both GluA1 and GluA2 (ref. 2 ). Our results were gathered using coimmunoprecipitation of endogenous proteins, a stringent and reliable method for assessing real protein-protein interaction. The data obtained were further confirmed by reverse coimmunoprecipitation—a method that is more likely to identify real protein interaction in in vivo systems. Therefore, we believe that our results are more accurate as the earlier techniques used to analyse protein interactions were likely less stringent. Collectively, our data are consistent with the model that GluA1 receptor is required for LTP and that SNX27 mediates the selective recruitment of homomeric GluA1 AMPARs to synapses. Earlier, GluA2-deficient mice were shown to exhibit enhanced LTP [32] and activity blockade was demonstrated to selectively enhance dendritic synthesis of GluA1 but not GluA2 (ref. 33 ); taken as a whole, our results underpin the selective importance of GluA1 subunit for AMPAR insertion during synaptic potentiation. Despite numerous studies on AMPARs in synaptic plasticity, the role of the C-terminal PDZ domain-binding motif of GluR1 in hippocampal LTP has been somewhat unclear. One model supports the idea that hippocampal LTP is independent of the GluA1 PDZ domain-binding motif [28] , [30] . The other equally plausible model is that synaptic accumulation of GluA1 containing AMPARs during LTP requires the interaction of GluA1 and a yet to be defined type I PDZ domain-containing protein, while synaptic incorporation of GluA2/GluA3 AMPARs occurs continuously and requires an interaction between GluA2 and a type II PDZ domain-containing protein [13] , [34] . Our results establish that SNX27, a Type I PDZ domain protein [1] , forms a complex with GluA1, but not GluA2 receptors, and identifies SNX27 as the type-I PDZ domain-containing protein important for the synaptic delivery of AMPARs. Since the early phase of LTP requires AMPAR insertion and is independent of protein synthesis, we employed a GluA1 optical reporter—engineered by fusing the N-terminal of AMPA GluA1 receptor with pH-sensitive GFP variant superecliptic pHluorin (SEP)—to directly assay the role of SNX27 in synaptic delivery of GluA1. Importantly, the results using chemical LTP stimuli on ectopically expressed GluA1 indicate that exocytosis of GluA1 was markedly diminished in the absence on SNX27. Thus during synaptic potentiation, CaM integrates the Ca 2+ -triggered plasticity signal and drives the translocation of K-ras to SNX27. We hypothesize that the binding of K-ras to SNX27 lowers the threshold for GluA1 insertion by promoting the critical ‘PDZ domain interaction’ between SNX27 and GluA1, thereby serving as a molecular gate that modulates AMPARs insertion during LTP. To examine the physiological importance of this result on synaptic plasticity, we measured LTP in the Schaffer collateral pathway. As expected, synaptic potentiation in physiological brain slices was completely abolished in the absence of SNX27, indicating that in the intact brain SNX27 is required for the induction of LTP. This result is consistent with a previous study which demonstrated that decreased LTP has been observed in SNX27+/−mice [2] . Therefore, a loss or reduction of SNX27 expression could account for memory impairments observed in pathologies where their levels are altered. Collectively, these results identify SNX27 as the novel activity-dependent signalling molecule that has the ability to decode the Ras signal and transduce the plasticity stimuli to the delivery of postsynaptic AMPARs. Since this study illustrates that SNX27 is important for the delivery of AMPA receptors during synaptic activity and Down’s syndrome is associated with the reduced expression of SNX27, this result could potentially account for the learning deficits observed in Down’s syndrome. Taken together, our biochemical, cell biological, physiological and genetic evidence suggests that SNX27 is likely the Type I PDZ domain protein previously implicated in the surface delivery of AMPARs associated with LTP. Constructs and antibodies SEP GluR1, mCherry-PSD95 and GFP-TfR were kindly provided by MD Ehlers (Duke University, North Carolina, USA). GFP-SNX27 and mCherry SNX27 were generated by subcloning human SNX27 (Origene) into pEGFP-N1 or pmCherry-N1 (Clontech) using Bgl11 and BamH1. The dilution and sources of the primary antibodies used were rabbit anti-GluA1 (1:100, AB31232), rabbit anti-GluA1(1:1,000, SYSY182-003), rabbit anti-GluA2 (1:1,000, SYSY 182-113), rabbit anti-GluN1(1:1,000, SYSY114-003), mouse anti-synaptophysin (1:50, AB8049), rabbit anti-K-ras (1:20, SC-30), rabbit anti-H-ras(1:200, SC-520), rabbit anti-N-ras(1:200, SC-519), mouse anti-Rab11 (1:100, transduction laboratories 610657), rabbit anti-SAP97(1:1,000, AB60551), rabbit anti-PSD95 (1:1,000, SYSY124-002), rabbit anti-HA (1:1,000, BethylA190-108A) and rabbit anti-myc (1:1,000, Upstate06-549). Full gel scans are provided in Supplementary Fig. 8 . Cell culture and transient transfection Hippocampal neuronal cultures were prepared from P0 mouse pups (mixed background 129/SV: C57BL6) and grown on 18-mm poly- D -lysine-coated coverslips at a density of 90 K per well in Neurobasal media/B27/Glutamax I without serum. One-third of the media was changed twice a week until use. Neurons were transfected using Lipofectamine 2000 (Invitrogen) according to the manufacturer’s recommendations. HEK293 cells were grown in DMEM supplemented with 10% fetal bovine serum and transfected using effectene reagent according to the manufacturer’s recommendations. Transferrin recycling assay Neurons were incubated with Alexa 568-Tf (50 μg ml −1 ) in serum-free Neurobasal media for 30 min at 37 °C to reach equilibrium. Neurons were then treated with or without glycine (200 μM) or glycine/APV in Neurobasal media for 25 min at room temperature. After washing, neurons were fixed and the remaining intracellular Alexa 568-Tf imaged. Live-cell imaging Live-cell imaging was performed on a custom-built spinning disk Confocal microscope with a Yokogawa CSU scan head mounted on a OlympusFV1000 inverted microscope. Twenty-four to 48 h following transfection, neurons were imaged in a chamber filled with extracellular solution containing in (mM): 130NaCl, 5KCl, 2CaCl 2 , 10HEPES, 30 glucose, 1 MgCl 2 (pH 7.4), using a × 60 Plan Apochromat objective (NA1.4) and the Photometrics Evolve EMCCD camera. Neurons were stimulated by exchanging the extracellular solution to one that contained (in mM): 130NaCl, 5KCl, 10 HEPES, 30 glucose, 3 CaCl 2 , 0.03(−) bicuculline methiodide, 0.2 glycine (pH 7.4, gly solution). The focal plane was controlled by a piezo-driven Z-stage (Applied Scientific Instruments). The EMCCD camera, filter wheel, stage and AOTF laser line switching were controlled by Metamorph software (Molecular Devices). An environmental chamber enclosing the microscope stand maintained the temperature at 37 °C. Preparation of synaptosomal and PSD fractions Mouse hippocampi were dissected and homogenized on ice in 10 volumes of cold sucrose buffer (0.32 M sucrose and 25 mM 4-(2-hydroxyethyl)-1-piperazineethanesulfonic acid (HEPES), pH 7.4). The homogenates were centrifuged at 300 g for 5 min to separate the supernatant (S1) from the nuclei and large debris fraction. The S1 fraction was centrifuged at 10,000 g for 12 min to separate the supernatant (S2; light membrane and cytosolic fraction) and the pellet (P2; crude synaptosomal fraction). The P2 fraction was washed twice with sucrose buffer and resuspended in cold HBS buffer (25 mM HEPES (pH 7.4) and 150 mM NaCl) to get the synaptosomal fraction. The Triton-insoluble fraction was prepared by solubilizing the synaptosomal fraction in 1% Triton HBS buffer at 4 °C for 30 min and then centrifuging at 10,000 g for 20 min. The Triton-insoluble (PSD) fraction was then solubilized in 2% SDS. CaM-binding assay HEK293 cells expressing HA-Kras, HA-Hras or HA-Nras were lysed in 150 mM NaCl, 50 mM Tris (pH 7.4) and 0.5% Triton X-100 in the presence of EDTA-free protease inhibitor cocktail (Roche) by passage through a 22G injection needle. After a 20-min spin at 13,000 r.p.m., the supernatant was incubated with CaM sepharose 4B beads (GE Healthcare) for 1 h at 4 °C in the presence of 1.3 mM Ca or 2 mM EGTA. Unbound material was removed by a quick centrifugation step. Beads were washed five times with wash buffer (150 mM NaCl, 50 mM Tris (pH 7.4) and 1% Triton X-100) and bound material was eluted by boiling beads in sample buffer. Electrophysiology Electrophysiological experiments were performed using transverse hippocampal slices cut from 4-week-old male SNX27 knockout/wild-type mice (eight pairs). Slices were equilibrated in oxygenated artificial cerebrospinal fluid (ACSF: NaCl 124 mM, KCl 4.8 mM, KH 2 PO 4 1.2 mM, CaCl 2 2 mM, MgSO 4 2 mM, NaHCO 3 26 mM and glucose 10 mM (pH 7.4)) at 31 °C for at least 2 h before being transferred to a submersion recording chamber (PSMI, Harvard Apparatus, Holliston, MA). The Schaffer collateral pathway was stimulated with a tungsten bipolar electrode (World Precision Instrument, USA) positioned in the stratum radiatum. Stimulus intensity was controlled by a constant current stimulus isolation unit (NL800, Warner Instruments, Hamden, CT), and stimulus timing was controlled by Clampex 10.3 software (Molecular Devices, Sunnyvale, CA, USA). fEPSP was recorded using a glass microelectrode (3–6 M) filled with 3 M NaCl and containing an Ag/AgCl wire, positioned in the stratum radiatum of CA1 ~1 mm away from the stimulus electrode. fEPSP were amplified 20 × , Bessel-filtered at 1 kHz and digitized at 10 kHz using a Multiclamp 700B amplifier and a Digidata 1440A digitizer (Molecular Devices, Sunnyvale, CA). At the start of each experiment, an input–output (I/O) curve was constructed. The stimulation pulse (0.2 ms duration, 0.05 Hz) selected for baseline measurement was adjusted to yield ~40% of its maximal slope for LTP recording. The stimulation pulse for baseline measurement was adjusted to yield ~70% of its maximal slope for LTD recording. After baseline responses had been stable for 20 min, LTP was induced using high-frequency stimulation at 100 Hz for 1 s (100 pulses). LTD was induced by low-frequency stimulation at 1 Hz for 15 min (900 pulses). How to cite this article: Loo, L. S. et al. A role for sorting nexin 27 in AMPA receptor trafficking. Nat. Commun. 5:3176 doi: 10.1038/ncomms4176 (2014).